The RAG2 C-terminus and ATM protect genome integrity by controlling antigen receptor gene cleavage Tight control of antigen-receptor gene rearrangement is required to preserve genome integrity and prevent the occurrence of leukaemia and lymphoma. Nonetheless, mistakes can happen, leading to the generation of aberrant rearrangements, such as Tcra/d – Igh inter-locus translocations that are a hallmark of ataxia telangiectasia-mutated (ATM) deficiency. Current evidence indicates that these translocations arise from the persistence of unrepaired breaks converging at different stages of thymocyte differentiation. Here we show that a defect in feedback control of RAG2 activity gives rise to bi-locus breaks and damage on Tcra/d and Igh in the same T cell at the same developmental stage, which provides a direct mechanism for generating these inter-locus rearrangements. Both the RAG2 C-terminus and ATM prevent bi-locus RAG-mediated cleavage through modulation of three-dimensional conformation (higher-order loops) and nuclear organization of the two loci. This limits the number of potential substrates for translocation and provides an important mechanism for protecting genome stability. B and T lymphocyte development is driven by V(D)J recombination, a process through which V, D and J gene-coding segments within each of the seven antigen receptor loci are rearranged to create a vast repertoire of antigen receptors [1] , [2] . Generation of receptor diversity through recombination is critical for shaping the adaptive arm of the immune system, enabling B and T cells to mount a focused and specific response to foreign antigen. This programmed rearrangement event relies on the lymphoid-specific proteins, RAG1 and RAG2 (recombination activating genes 1 and 2), which individually harbour many distinct regulatory domains whose functions remain largely enigmatic. Nonetheless, it is known that at least some of these contribute to the performance of RAG through fine-tuning of targeting, cleavage and repair. Furthermore, the proper functioning of the recombinase complex relies on cooperation between the two proteins, RAG1 and 2. Specificity of targeting is conferred by RAG1-mediated recognition of highly conserved recombination signal sequence (RSS) elements that flank the individual V, D and J gene-coding segments, which are arrayed along each antigen receptor locus [3] , [4] , [5] . Moreover, RAG1 carries the catalytic endonuclease activity [4] , [5] . However, cleavage cannot occur in the absence of its partner protein, RAG2 (refs 6 , 7 ), which contains a plant homeo domain that is known to directly bind the recombinase to active chromatin through recognition of the histone modification, H3K4me3 (refs 8 , 9 ). The RAG1/2 complex binds to two gene segments (that can be many kilobases apart), brings them together and cuts at the RSS borders to generate DNA double-strand breaks (DSBs). Following cleavage, the four resulting broken ends are held together in a RAG post-cleavage complex that is instrumental in directing repair by the ubiquitous non-homologous end joining pathway [1] , [2] , [10] , [11] . The introduction of DSBs activates several PI3K-like Ser/Thr kinases, including the ataxia telangiectasia-mutated (ATM) kinase, which phosphorylate downstream proteins and orchestrate the DNA-damage response [2] . Other DNA-damage response factors, like the histone variant γ-H2AX, 53BP1 (p53-binding protein 1) and the MRN complex (containing Mre11, Rad50 and Nbs1), are rapidly recruited and form nuclear foci at the site of DSBs [2] , [11] . Recombination is tightly regulated so that the appropriate loci and gene segments are rearranged in the appropriate lineage (T-cell receptor ( Tcr ) loci in T cells and immunoglobulin ( Ig ) loci in B cells) and at the appropriate developmental stage. In T cells, productive rearrangement of the different Tcr loci gives rise to two distinct lineages: recombination of Tcrg / Tcrd and Tcrb/Tcra leads to γδ- and αβ-T cells, respectively [12] , [13] . Despite this separation, recombination of the different loci overlaps. Tcrg , Tcrd and Tcrb are all rearranged at the early CD4 − CD8 − double-negative (DN) 2/3 stage of development, whereas Tcra recombination occurs later in double-positive (DP) cells [14] . Regulation of Tcrd and Tcra recombination is uniquely complicated because, beyond the fact that they recombine at different stages of differentiation, Tcra and Tcrd share the same chromosomal location, with the latter embedded between the Vα and Jα gene segments. Furthermore, promiscuous D H to J H rearrangement of the Igh locus, which occurs at low level in T-lineage cells [15] , adds yet another layer of complexity. Together, these issues compound the risks associated with Tcra/d recombination and the probability of aberrant repair. Indeed, inter-locus rearrangements between Tcra/d and Igh have been identified as a hallmark of thymic lymphomas in ATM-deficient mice [16] . Moreover, we recently discovered translocations between these two loci associated with an absence of the non-core C-terminal domain of RAG2 (ref. 17 ). Although this domain is dispensable for recombination [18] , [19] , its deletion is known to affect the joining step, as well as the order, efficiency and fidelity of the reaction [10] , [20] , [21] , [22] , [23] , [24] , [25] . When coupled with the disruption of p53, we found that Rag2 c/c p53 −/− mice develop thymic lymphomas harbouring recurrent translocations involving Tcra/d and Igh , defects that are similar to those found in Atm −/− mice [17] . In addition, ATM and the C-terminus of RAG2 have similar defects in stabilizing the RAG post-cleavage complex [17] , [26] . Here we have now investigated the mechanisms underlying the origins of the inter-locus Igh – Tcra/d translocations before lymphomagenesis to determine whether regulation of cleavage and nuclear accessibility of the loci is perturbed by an absence of ATM and the C-terminus of RAG2. We find that Igh cleavage occurs at higher levels in DN2/3 versus DP cells, and thus its rearrangement could overlap with Tcra/d rearrangement. However, breaks are not found in Igh and Tcra/d in the same cell, except in the absence of the RAG2 C-terminus or ATM. Control of mono-locus cleavage involves regulated mono-locus looping out from the chromosome territory and mono-locus association with repressive pericentromeric heterochromatin (PCH). In the absence of the RAG2 C-terminus or ATM, nuclear accessibility is increased and both loci remain euchromatic, and bi-locus loops can be detected coincident with bi-locus cleavage. Interestingly, we found that expression of RAG brings Tcra/d and Igh into close proximity in DN2/3 cells (when RAG-mediated cleavage of Igh occurs at high levels), whereas the two loci separate at the subsequent DP cell stage of development (when recombination of Igh is reduced). In contrast, in the mutant cells, increased association of Tcra/d - Igh in DP cells is linked to increased nuclear accessibility, and the introduction of bi-locus breaks and damage on proximal loci. In sum, this study show a role for the non-core domain of RAG2 and ATM in controlling recombination between two loci via modulation of nuclear organization. Moreover, these events provide a direct mechanism for the generation of the Tcra/d - Igh translocations that are found in Rag2 c/c p53 −/− and Atm −/− tumours. Igh and Tcra/d rearrangement overlaps in DN2/3 and DP cells Although it is established that the Igh locus (which is located on chromosome 12) undergoes low-level D H –J H rearrangement (at the 3′ end of the locus) in T cells, it is not known at which stage of development recombination occurs. To determine this, we performed an immuno-DNA fluorescence in situ hybridization (FISH) experiment to analyse RAG-mediated cleavage on Igh in wild-type DN2/3 and DP cells ( Fig. 1a ) using a DNA probe that hybridizes to the 3′ end of this locus (see Fig. 1b ) in combination with an antibody against the phosphorylated form of H2AX, γ-H2AX, as a read-out for double-stranded breaks (DSBs) [27] , [28] . Our analyses showed that RAG-mediated γ-H2AX foci were associated more frequently with Igh in DN2/3 compared with DP cells, suggesting that D H –J H rearrangement occurs predominantly, but not exclusively, at the earlier stage of development ( Fig. 1c and Supplementary Table S1 ). In contrast, RAG-mediated γ-H2AX foci were associated more frequently with Tcra/d in DP compared with DN2/3 cells ( Fig. 1c and Supplementary Table S1 ). 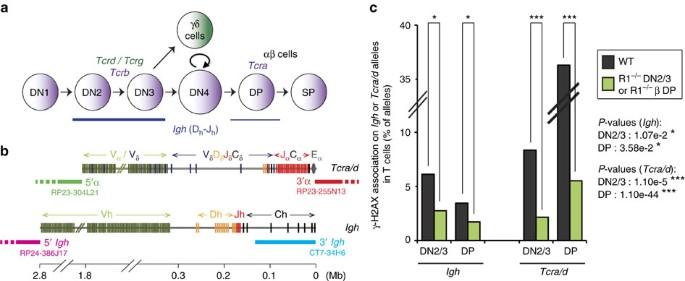Figure 1:IghandTcra/drearrangement overlaps in DN2/3 and DP T cells. (a) Scheme of T-cell development with stages of recombination of the fourTcrloci. (b) Scheme representing theTcra/dandIghloci with probes for 3D DNA FISH shown below. (c) Frequency of γ-H2AX association onIghorTcra/dalleles in wild-type (WT) DN2/3 and DP cells.P-values were calculated using a two-tail Fisher’s exact test, *significant (5.00e-2>P≥1.00e-2) and ***highly significant (P<1.00e-3)). Experiments were repeated at least two times, and data are displayed as a combination of two independent experimental sets (n>500 for each stage/genotype; seeSupplementary Table S1for details and individual data sets). Figure 1: Igh and Tcra/d rearrangement overlaps in DN2/3 and DP T cells. ( a ) Scheme of T-cell development with stages of recombination of the four Tcr loci. ( b ) Scheme representing the Tcra/d and Igh loci with probes for 3D DNA FISH shown below. ( c ) Frequency of γ-H2AX association on Igh or Tcra/d alleles in wild-type (WT) DN2/3 and DP cells. P -values were calculated using a two-tail Fisher’s exact test, *significant (5.00e-2> P ≥1.00e-2) and ***highly significant ( P <1.00e-3)). Experiments were repeated at least two times, and data are displayed as a combination of two independent experimental sets ( n >500 for each stage/genotype; see Supplementary Table S1 for details and individual data sets). Full size image The RAG2 C-terminus and ATM regulate mono-locus cleavage As both Tcra/d and Igh loci undergo recombination in T cells, it is conceivable that there is an overlap in the timing of their rearrangement. If so, bi-locus breaks could be introduced concurrently in the same cell, and, in the event of a defect in joining, these could act as substrates for translocations. However, when we examined the frequency of γ-H2AX foci associated with both Tcra/d and Igh (bi-locus breaks) in individual wild-type DN2/3 and DP cells, we found these present at a very low level, which was only slightly above the frequency of bi-locus breaks detected in RAG-deficient cells ( Fig. 2a and Supplementary Tables S2 and S3 ). In contrast, we found a significant rise in the frequency of bi-locus breaks in individual Rag2 c/c p53 −/− or Atm −/− cells, with the most pronounced increase occurring at the DP stage, at the time of Tcra recombination ( Fig. 2a,b and Supplementary Tables S2 and S3 ). It is of note that we found no increase in the frequency of bi-locus breaks in the absence of another DNA-damage response factor, 53BP1, which is known to be important for the long-range joining of coding ends in V(D)J recombination [29] ( Fig. 2a and Supplementary Tables S2 and S3 ). These data indicate that bi-locus breaks in the same cell do not occur simply as a result of a defect in repair. 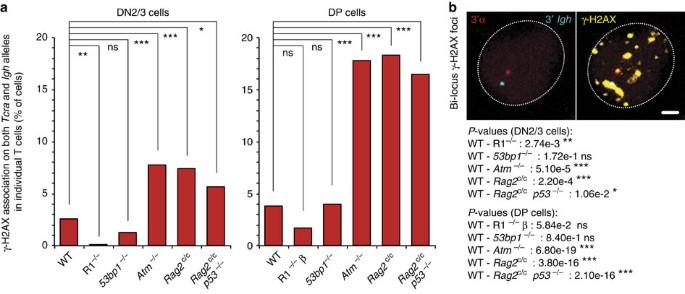Figure 2: The RAG2 C-terminus and ATM regulate mono-locus cleavage. (a) Frequency of γ-H2AX association on bothTcra/dandIghloci in individual wild-type (WT),Rag1−/−(R1−/−or R1−/−β (see Methods section for details)),53bp1−/−,Atm−/−,Rag2c/candRag2c/cp53−/−DN2/3 and DP cells. (b) Confocal sections showing a representative example of γ-H2AX association (in yellow) on bothTcra/dandIghloci (3′α in red, 3′Ighin blue). Scale bar, 1 μm.P-values were calculated using a two-tail Fisher’s exact test (ns, no significance (P≥5.00e-2), *significant (5.00e-2>P≥1.00e-2), **very significant (1.00e-2>P≥1.00e-3) and ***highly significant (P<1.00e-3)). Experiments were repeated at least two times, and data are displayed as a combination of two independent experimental sets (n>200 for each stage/genotype; seeSupplementary Tables S2 and S3for details and individual data sets). Figure 2: The RAG2 C-terminus and ATM regulate mono-locus cleavage. ( a ) Frequency of γ-H2AX association on both Tcra/d and Igh loci in individual wild-type (WT), Rag1 −/− (R1 −/− or R1 −/− β (see Methods section for details)), 53bp1 −/− , Atm −/− , Rag2 c/c and Rag2 c/c p53 −/− DN2/3 and DP cells. ( b ) Confocal sections showing a representative example of γ-H2AX association (in yellow) on both Tcra/d and Igh loci (3′α in red, 3′ Igh in blue). Scale bar, 1 μm. P -values were calculated using a two-tail Fisher’s exact test (ns, no significance ( P ≥5.00e-2), *significant (5.00e-2> P ≥1.00e-2), **very significant (1.00e-2> P ≥1.00e-3) and ***highly significant ( P <1.00e-3)). Experiments were repeated at least two times, and data are displayed as a combination of two independent experimental sets ( n >200 for each stage/genotype; see Supplementary Tables S2 and S3 for details and individual data sets). Full size image Because cells deficient in both p53 and ATM have defects in cell cycle checkpoints that enable unrepaired breaks to be propagated as a result of cell division [30] , [31] , it is possible that some proportion of the bi-locus breaks that we detected in mutant DP cells could be attributed to the persistence of unrepaired breaks being amplified in proliferating DN4 cells, which mark the transition from the DN2/3 to the DP stage of development ( Fig. 1a ). To check this, we compared the frequency of bi-locus breaks in individual Rag2 c/c versus Rag2 c/c p53 −/− cells. However, we found no significant differences in the incidence of bi-locus breaks in the two genotypes, and so we conclude that the increase in bi-locus breaks that we detected in Rag2 c/c p53 −/− DP cells does not result from an absence of p53 ( Fig. 2a and Supplementary Tables S2 and S3 ). Indeed, we also found no significant increase in bi-locus breaks on Tcra/d and Igh in wild-type versus p53 −/− cells (4% versus 4.6%, respectively). In addition, differences in the level of ATM in Rag2 c/c versus wild-type cells cannot explain the differences in the frequency of bi-locus breaks, as western blot analysis showed similar levels of protein in the two genotypes ( Supplementary Fig. S1 ). Taken together, these data indicate that the C-terminus of RAG2 and ATM regulate cleavage to ensure that RAG-mediated breaks are introduced on only one locus at a time in each recombining T cell. The RAG2 C-terminus and ATM regulate Tcra – Igh association We and others have shown that nuclear proximity of broken partner genes is an important factor in translocations [32] , [33] , [34] , [35] , [36] , [37] . As our studies indicate that translocations between Tcra/d and Igh are found in tumours from Rag2 c/c p53 −/− and Atm −/− mice [17] , we wanted to examine the association between the two loci in recombining DN2/3 and DP cells. For this, we performed circularized chromosome conformation capture with next-generation sequencing (4C-seq), using a bait sequence spanning the Tcra enhancer (Eα) at the 3′α end of the locus (see Methods section for details; Fig. 3a , Supplementary Fig. S2a and Supplementary Table S4 ). The 4C data are displayed as a domainogram, which is a statistical way to visualize local 4C signal enrichment across a region of interest [38] . It is clear from Fig. 3a (left panels) that there are significant changes in the interaction partners of Tcra/d in the two populations across chromosome 12. Importantly, the intensity of the Tcra / d – Igh interaction is much higher in DN2/3 cells where, according to our γ-H2AX analysis, the latter is recombined at higher frequency ( Fig. 3a (right panels)). This result was validated by additional three-dimensional (3D) DNA FISH experiments, and distances separating the two loci were plotted as cumulative frequency curves, using a cut-off of 1 μm to measure close association (that is, ‘pairing’) ( Supplementary Fig. S2b ). On these graphs, a left shift is indicative of closer association. Examples of paired and unpaired loci are shown in Fig. 3b . 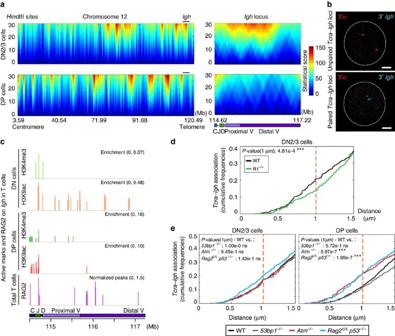Figure 3: The RAG2 C-terminus and ATM regulateTcra–Ighassociation. (a) Domainograms showing a heatmap ofTcra/dinteractions across the entire chromosome 12 (left) and theIghlocus (right) using a window size of 30HindIII sites in DN2/3 (top) and DP (bottom) cells. See alsoSupplementary Fig. S2andSupplementary Table S4. (b) Confocal sections showing representative examples of unpaired (top) and paired (bottom) loci: 3′α in red, 3′Ighin blue. Scale bars, 1 μm. (c) Alignment of ChIP-seq data at theIghlocus showing levels of enrichment of H3K4me3 (green), H3K9ac (red) and RAG2 binding (purple)39in DN and DP cells. See alsoSupplementary Table S5. (d,e) Cumulative frequency curves ofTcra–Ighinter-locus distances in: wild-type (WT) and R1−/−DN2/3 cells (d), WT,53bp1−/−,Atm−/−andRag2c/cp53−/−DN2/3 (e, left) and DP (e, right) cells (cut-off at 1.5 μm). A left shift indicates closer association.P-values were calculated using a two-tail Fisher’s exact test (ns, no significance (P≥5.00e-2) **very significant (1.00e-2>P≥1.00e-3) and ***highly significant (P<1.00e-3)). Experiments were repeated at least two times, and data are displayed as a combination of two independent experimental sets (n>200 for each stage/genotype). Figure 3: The RAG2 C-terminus and ATM regulate Tcra – Igh association. ( a ) Domainograms showing a heatmap of Tcra/d interactions across the entire chromosome 12 (left) and the Igh locus (right) using a window size of 30 Hin dIII sites in DN2/3 (top) and DP (bottom) cells. See also Supplementary Fig. S2 and Supplementary Table S4 . ( b ) Confocal sections showing representative examples of unpaired (top) and paired (bottom) loci: 3′α in red, 3′ Igh in blue. Scale bars, 1 μm. ( c ) Alignment of ChIP-seq data at the Igh locus showing levels of enrichment of H3K4me3 (green), H3K9ac (red) and RAG2 binding (purple) [39] in DN and DP cells. See also Supplementary Table S5 . ( d , e ) Cumulative frequency curves of Tcra – Igh inter-locus distances in: wild-type (WT) and R1 −/− DN2/3 cells ( d ), WT, 53bp1 −/− , Atm −/− and Rag2 c/c p53 −/− DN2/3 ( e , left) and DP ( e , right) cells (cut-off at 1.5 μm). A left shift indicates closer association. P -values were calculated using a two-tail Fisher’s exact test (ns, no significance ( P ≥5.00e-2) **very significant (1.00e-2> P ≥1.00e-3) and ***highly significant ( P <1.00e-3)). Experiments were repeated at least two times, and data are displayed as a combination of two independent experimental sets ( n >200 for each stage/genotype). Full size image Previous studies indicate that RAG binds to active chromatin and localizes to the J segments at the 3′ end of each antigen receptor locus in rearranging cells [39] . We have recently shown that localized RAG enrichment in this region is linked with homologous Tcra pairing, transcription and regulated mono-allelic cleavage in DP cells [40] . Thus, we wanted to investigate whether the presence of RAG could influence the frequency with which Tcra/d and Igh contact each other during recombination. There are two regions of RAG2 binding on the Igh locus in developing T cells ( Fig. 3c ). The first corresponds to enrichment of H3K4me3 and H3K9ac at the 3′ end of Igh , where D H –J H rearrangement is known to occur in these cells [15] . In addition, RAG2 also binds to the V H portion of Igh , and this could explain the high frequency of interaction with Tcra in this region ( Fig. 3a,c and Supplementary Table S5 ). Interestingly, we found that an absence of RAG1 significantly decreased heterologous association of the two loci in DN2/3 cells, whereas we observed no significant change in DP cells ( Fig. 3d and Supplementary Fig. S2c ). These data indicate that RAG1 brings recombining Tcra/d and Igh together in DN2/3 cells (where Igh cleavage occurs at high levels) but that these loci separate in DP cells (where cleavage of Igh is reduced and cleavage of Tcra occurs at high levels) ( Fig. 1c ). Intriguingly, the absence of the C-terminus of RAG2 or ATM deficiency did not affect the frequency of Tcra / d-Igh association in DN2/3 cells; however, in DP cells, where association of the two loci is normally reduced, we observed an increase in the incidence of heterologous pairing in both mutants, although pairing in the equivalent 53BP1-deficient populations followed the same pattern as in wild-type cells ( Fig. 3e ). Importantly, bi-locus breaks were increased on heterologously paired loci in Rag2 c/c p53 −/− and Atm −/− DP cells compared with wild-type control and 53BP1-deficient cells ( Fig. 4a,b and Supplementary Table S6 ). These data indicate that an increased frequency in contact between Tcra and Igh in Rag2 c/c p53 −/− and Atm −/− DP cells is linked to an increased frequency in bi-locus breaks on paired loci. 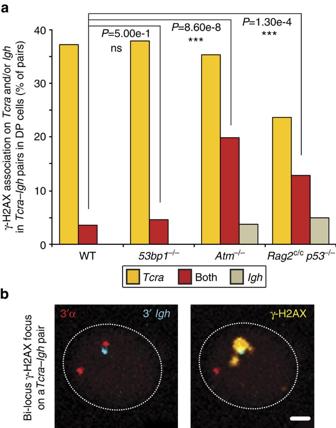Figure 4: RAG2 C-terminus and ATM control cleavage onTcra–Ighpairs. (a) Frequency of γ-H2AX association onTcraand/orIghinTcra–Ighpairs in wild-type (WT),53bp1−/−,Atm−/−andRag2c/cp53−/−DP cells. (b) Confocal sections showing a representative example of aTcra–Ighpair with a γ-H2AX focus on both loci. 3′α in red, 3′Ighin blue and γ-H2AX in yellow. Scale bar, 1 μm.P-values were calculated using a two-tail Fisher’s exact test (ns, no significance (P≥5.00e-2), ***highly significant (P<1.00e-3)). Experiments were repeated at least two times, and data are displayed as a combination of two independent experimental sets (n>80 for each genotype; seeSupplementary Table S6for details and individual data sets). Figure 4: RAG2 C-terminus and ATM control cleavage on Tcra–Igh pairs. ( a ) Frequency of γ-H2AX association on Tcra and/or Igh in Tcra–Igh pairs in wild-type (WT), 53bp1 −/− , Atm −/− and Rag2 c/c p53 −/− DP cells. ( b ) Confocal sections showing a representative example of a Tcra–Igh pair with a γ-H2AX focus on both loci. 3′α in red, 3′ Igh in blue and γ-H2AX in yellow. Scale bar, 1 μm. P -values were calculated using a two-tail Fisher’s exact test (ns, no significance ( P ≥5.00e-2), ***highly significant ( P <1.00e-3)). Experiments were repeated at least two times, and data are displayed as a combination of two independent experimental sets ( n >80 for each genotype; see Supplementary Table S6 for details and individual data sets). Full size image RAG-mediated pairing is not a general phenomenon Genome-wide analysis has shown that RAG2 has an overlapping pattern with H3K4me3-enriched regions [39] ; thus, we wanted to determine whether other RAG-enriched active genes would pair up with Tcra in the same way as Igh. For this analysis, we selected five hematopoietic lineage-specific genes ( Hmgb1 , Lat , Cd3g , Ly6d and Satb1 ), as well as a housekeeping gene ( Gapdh ), which are all located on different chromosomes and transcribed in these cells ( Fig. 5a,b ). Interestingly, pairing of Tcra with these other RAG-enriched loci shows an opposite trend to Igh – Tcra pairing in all cases ( Fig. 5c and Supplementary Table S7 ). Indeed, in contrast to Tcra – Igh , an absence of RAG1 appears to increase their contact frequency with Tcra in DN2/3 cells, and association is even more pronounced at the DP stage of development. Furthermore, pairing between these control loci follows the same trend as their association with Tcra ( Fig. 5d and Supplementary Table S7 ). It is of note that the maximum frequency of pairing (for individual pairs of alleles) in all cases is very similar (around 20%), and this matches the maximum level of homologous Tcra pairing seen during recombination in DP cells [40] . Taken together, these data indicate that the trend for Tcra – Igh is unique, and even though RAG2 is enriched on control loci, pairing does not depend on the presence of RAG. Instead, interactions between control loci may be influenced by binding of other transcription factors that are involved in their regulation. In this context, the Fraser lab has shown that co-ordinately regulated genes associate with each other in common transcription factories, and more recent studies from the Murre lab indicate that transcription-factor-bound regions determine intra- and inter-domain interactions that are developmentally regulated [41] . Thus, perhaps other transcription factors that are enriched on these control genes may be dominant in determining their interaction partners in developing T-cell nuclei. 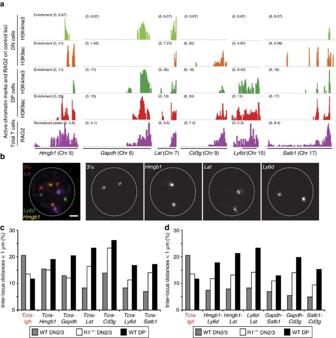Figure 5: RAG-mediated pairing is not a general phenomenon. (a) Alignment of ChIP-seq data at theHmgb1,Gapdh,Lat,Cd3g,Ly6dandSatb1loci showing levels of enrichment of H3K4me3 (green), H3K9ac (red) and RAG2 binding (purple)39in DN and DP cells. (b) Confocal sections showing 3D DNA FISH forTcraand three control loci. 3′α in red,Hmgb1in yellow,Latin purple andLy6din green. Scale bar, 1 μm. (c,d) Graphs showing the frequency of heterologous pairing (inter-locus distance <1 μm) betweenTcraand the control loci (c), or between the loci (d). Experiments were performed at least one time, and data are displayed as a combination of independent experimental sets when applicable (n>200 for each stage/genotype; seeSupplementary Table S7for details). Figure 5: RAG-mediated pairing is not a general phenomenon. ( a ) Alignment of ChIP-seq data at the Hmgb1 , Gapdh , Lat , Cd3g , Ly6d and Satb1 loci showing levels of enrichment of H3K4me3 (green), H3K9ac (red) and RAG2 binding (purple) [39] in DN and DP cells. ( b ) Confocal sections showing 3D DNA FISH for Tcra and three control loci. 3′α in red, Hmgb1 in yellow, Lat in purple and Ly6d in green. Scale bar, 1 μm. ( c , d ) Graphs showing the frequency of heterologous pairing (inter-locus distance <1 μm) between Tcra and the control loci ( c ), or between the loci ( d ). Experiments were performed at least one time, and data are displayed as a combination of independent experimental sets when applicable ( n >200 for each stage/genotype; see Supplementary Table S7 for details). Full size image Regulation of RAG cleavage is linked to genome stability The Tcra and Igh loci are located on different chromosomes, namely chromosomes 14 and 12, respectively. To understand how association between these two loci occurs in nuclear space, we focused our attention on the formation of higher-order loops that move genes outside of their chromosome territories as a mechanism by which they could be brought into close contact. We recently showed that mono-locus looping out of Tca is linked to homologous pairing during recombination [40] . To examine this, we measured the distance separating the 3′ end of Tcra and Igh from their respective chromosome 14 and 12 territories when the loci were paired. Our analyses indicate that in wild-type DP cells the vast majority of higher-order loop formation occurred on one locus at a time, and these predominantly involved Tcra ( Fig. 6a,b and Supplementary Table S8 ), the locus in which we detected the most breaks ( Fig. 4a ). In contrast, there was a significant increase in bi-locus loop formation on paired Tcra – Igh alleles in Rag2 c/c p53 −/− and Atm −/− DP cells ( Fig. 6a,b and Supplementary Table S8 ), coincident with an increase in bi-locus breaks ( Fig. 4a ). Taken together, our data indicate that an increase in Tcra – Igh pairing in Rag2 c/c p53 −/− and Atm −/− DP cells is linked to an increase in bi-locus looping and bi-locus breaks on paired alleles. 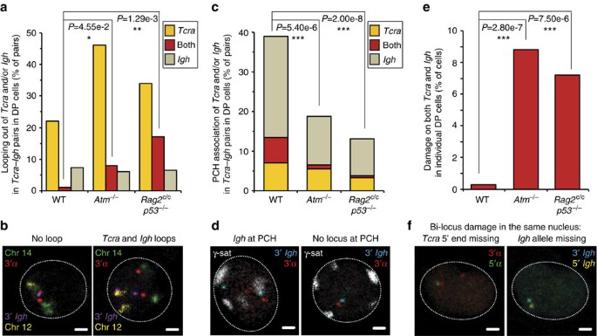Figure 6: Regulation of RAG cleavage is linked to genome stability. (a) Frequency of higher-order looping out of the 3′ ends ofTcraand/orIghinTcra–Ighpairs in wild-type (WT),Atm−/−andRag2c/cp53−/−DP cells. (b) Confocal sections showing examples ofTcra–Ighpairs with no loop or looping of bothTcraandIgh. 3′α in red, 3′Ighin purple, chromosome 14 in green and chromosome 12 in yellow. Scale bars, 1 μm. (c) Frequency of PCH association ofTcraand/orIghinTcra–Ighpairs in WT,Atm−/−andRag2c/cp53−/−DP cells. (d) Confocal sections showing representative examples ofTcra–Ighpairs withIghlocated at PCH or no locus at PCH. 3′α in red, 3′Ighin blue and γ-satellite (PCH) in white. Scale bars, 1 μm. (e) Frequency of cells with bi-locus damage on bothTcra/dandIghalleles in individual WT,Atm−/−andRag2c/cp53−/−DP cells. (f) Confocal sections showing a representative example of bi-locus damage on bothTcraandIghalleles in the same nucleus. OneTcra5′ end and oneIghallele are missing. 3′α in red, 5′α in green, 3′Ighin blue and 5′Ighin yellow. Scale bars, 1 μm.P-values were calculated using a two-tail Fisher’s exact test (ns, no significance (P≥5.00e-2), *significant (5.00e-2>P≥1.00e-2), ** very significant (1.00e-2>P≥1.00e-3) and ***highly significant (P<1.00e-3)). Experiments were repeated at least two times, and data are displayed as a combination of two independent experimental sets (n>50 for each genotype; seeSupplementary Tables S8–S10for details). Figure 6: Regulation of RAG cleavage is linked to genome stability. ( a ) Frequency of higher-order looping out of the 3′ ends of Tcra and/or Igh in Tcra–Igh pairs in wild-type (WT), Atm −/− and Rag2 c/c p53 −/− DP cells. ( b ) Confocal sections showing examples of Tcra–Igh pairs with no loop or looping of both Tcra and Igh . 3′α in red, 3′ Igh in purple, chromosome 14 in green and chromosome 12 in yellow. Scale bars, 1 μm. ( c ) Frequency of PCH association of Tcra and/or Igh in Tcra–Igh pairs in WT, Atm −/− and Rag2 c/c p53 −/− DP cells. ( d ) Confocal sections showing representative examples of Tcra–Igh pairs with Igh located at PCH or no locus at PCH. 3′α in red, 3′ Igh in blue and γ-satellite (PCH) in white. Scale bars, 1 μm. ( e ) Frequency of cells with bi-locus damage on both Tcra/d and Igh alleles in individual WT, Atm −/− and Rag2 c/c p53 −/− DP cells. ( f ) Confocal sections showing a representative example of bi-locus damage on both Tcra and Igh alleles in the same nucleus. One Tcra 5′ end and one Igh allele are missing. 3′α in red, 5′α in green, 3′ Igh in blue and 5′ Igh in yellow. Scale bars, 1 μm. P -values were calculated using a two-tail Fisher’s exact test (ns, no significance ( P ≥5.00e-2), *significant (5.00e-2> P ≥1.00e-2), ** very significant (1.00e-2> P ≥1.00e-3) and ***highly significant ( P <1.00e-3)). Experiments were repeated at least two times, and data are displayed as a combination of two independent experimental sets ( n >50 for each genotype; see Supplementary Tables S8–S10 for details). Full size image Higher-order looping of genes away from their chromosome territories has previously been correlated with open chromatin and an active transcriptional status, while silent genes are positioned more internally [43] , [44] , [45] , [46] . To determine whether nuclear accessibility of the individual loci is linked to loop formation, we examined the location of paired Tcra–Igh relative to the repressive pericentromeric heterochromatin (PCH). In wild-type DP cells, we found that paired Tcra–Igh alleles were frequently located at PCH; however, the two loci were not equivalently close ( Fig. 6c,d and Supplementary Table S9 ). Interestingly, we found that the Igh locus was predominantly in contact with PCH, whereas Tcra , the locus associated with the most loops and breaks in these pairs, remained euchromatic. In contrast, in Rag2 c/c p53 −/− and Atm −/− DP cells, repositioning of the Igh to PCH was significantly reduced, and this increased nuclear accessibility was associated with increased bi-locus breaks ( Fig. 6c,d ). These data indicate that the increase in bi-locus breaks on paired Tcra – Igh alleles in Rag2 c/c p53 −/− and Atm −/− DP cells is linked with an increase in the simultaneous nuclear accessibility of the two loci, as assessed by looping out from their chromosome territories and by their location away from repressive PCH. Because close proximity of broken partner loci in DP cells could provide a fertile ground for the generation of the aberrant inter-locus rearrangements that are a characteristic of Rag2 c/c p53 −/− and Atm −/− lymphomas, we next asked whether the increase in bi-locus breaks and increased accessibility of paired Tcra/d / Igh was linked with an increase in bi-locus instability in interphase Rag2 c/c p53 −/− and Atm −/− cells before the onset of lymphomagenesis. For this, we performed a DNA FISH experiment using DNA probes that hybridize outside the 3′ and 5′ ends of each locus (see Fig. 1b ) and examined the frequency of damage (that is, split alleles (>1.5 μm in between the two ends), duplicated or missing signals). The increase in bi-locus damage in individual Rag2 c/c p53 −/− - and Atm −/− -mutant DP cells was very significant ( Fig. 6e,f and Supplementary Table S10 ). Thus, an absence of the C-terminal domain of RAG2 or ATM results in an increase in both bi-locus breaks and bi-locus damage in the same cell. Taken together, our data show that translocations between Tcra/d and Igh that are found in tumours from Rag2 c/c p53 −/− and Atm −/− mice [17] may arise not only as a result of Tcrd recombination (as shown previously in ATM-deficient mice [16] ) but also from Tcra recombination. It has previously been proposed that the aberrant inter-locus Tcra/d – Igh rearrangements found in Atm −/− T cells arise from the persistence of unrepaired breaks converging at different stages of thymocyte differentiation [16] . However, in contrast to our analyses, these studies did not examine breaks on Tcra/d and Igh in individual developing T cells, but rather they analysed translocations in Atm −/− mature T cells and Atm −/− -derived thymic lymphomas, respectively. Here we show that breaks on the two loci occur in the same cell at the same stage of development, which provides a direct mechanism for the generation of the characteristic inter-locus Tcra/d – Igh translocations that are found in Rag2 c/c p53 −/− and Atm −/− [17] , [47] , [48] T lymphomas. Our studies reveal that there is similarity between the C-terminus of RAG2 and ATM in temporally harnessing RAG activity to ensure that cleavage occurs on only one locus at a time in recombining T cells. Intriguingly, we find that RAG-mediated association of recombining loci in localized ‘recombination centres’ is linked to feedback control of RAG cleavage: the introduction of a break on one locus is coupled with repositioning of the partner locus to PCH and inhibition of bi-locus cleavage and looping out from the territory (see Model in Supplementary Fig. S3 ). Targeting of RAG to the correct locus ( Tcra rather than Igh ) is likely to be influenced by the higher level of transcription on Tcra. Interestingly, although cleavage of Tcra is reduced in paired Tcra/d – Igh alleles in Rag2 c/c p53 −/− DP cells (perhaps due to a decrease in efficiency of cleavage in the absence of the C-terminus of RAG2), there is a significant increase in cleavage of Igh , which further underlines the role of regulation in trans between the two loci. Although we recently showed that pairing and higher-order looping of Tcra homologous alleles are linked with regulation of their recombination [40] , cross-talk and regulation of heterologous loci in trans have not previously been shown to be linked to the formation of higher-order looping. Indeed, higher-order loop formation was previously shown to be involved in stochastic interactions between different loci on separate chromosomes [41] , [49] , although we have found here that interactions between Tcra/d and Igh are mediated by the presence of RAG. Together, our data suggest that regulation of mono-locus cleavage relies on changes in nuclear organization that are associated with a reduction in accessibility. Regulation of mono-locus cleavage is thus akin to regulation of mono-allelic cleavage. Indeed, our previous studies showed that ATM recruited to the site of a break on one allele acts in trans to reposition the second homologous allele to PCH and to prevent the introduction of further breaks on the partner homologue [40] , [50] . We propose that homologous and heterologous antigen receptor alleles come together in localized recombination centres for coordinated regulation of RAG cleavage. Here we have now identified an auto-regulatory role for RAG2 in restricting cleavage in an analogous manner to ATM. These data explain the mechanisms underlying the origins of the inter-locus Igh – Tcra/d in Atm −/− and Rag2 c/c p53 −/− lymphocytes before lymphomagenesis. Importantly, they identify an unappreciated role for the C-terminal domain of RAG2 in regulating chromosome dynamics and accessibility of target loci to restrict ongoing cleavage after the introduction of a break on one locus. Thus, feedback control of RAG activity relies on signals transmitted via the RAG complex itself. Regulation of V(D)J recombination occurs at multiple levels to prevent the occurrence of chromosomal translocations or deletions that can result from errors in repair and/or mis-targeting of RAG1/2 to cryptic RSSs. However, beyond degradation of RAG2 protein [51] and our more recent findings that expression of Rag1 is regulated across cell cycle [52] , there been have no studies that focus specifically on autoregulation of RAG cleavage activity in individual cells. It is clearly critical to have such mechanisms in place to ensure that further breaks are not introduced in cis or trans on accessible target loci that undergo recombination at overlapping stages of development ( Tcrg , Tcrb , Tcrd and Igh in DN T cells and Igk and Igl in pre-B/immature B cells). Furthermore, this same mechanism could also be important in preventing cleavage on actively transcribed off-target loci with cryptic RSSs that bind RAG. Mice The Atm −/− , Rag2 c/c and Rag2 c/c p53 −/− mice were provided by Deriano et al. [17] RAG1-deficient mice were provided by Yanhong Ji, Grace Teng and David Schatz: RAG1-deficient DP cells (R1 −/− -β and control WT-β) were derived from mice carrying a functionally rearranged Tcrb transgene (β) that allows T-cell development to proceed to the DP stage in the absence of Tcrb rearrangement. The 53BP1 −/− mice were provided by Davide Robbiani and Michel Nussenzweig [53] . Wild-type littermates were used as controls. Animal care was approved by the NYU School of Medicine Animal Care and Use Committee of (protocol number 120315-01). T-cell flow-cytometry sorting Flow-cytometry cell sorting was performed on a MoFlo or Reflection sorter. Antibodies were as follows: Thy1.2 PE-Cy7 (CD90.2, clone 53-2.1, 1:1,000 dilution; eBioscience), TCRβ APC-eFluor780 (clone H57-597, 1:500 dilution; eBioscience), CD4 APC (L3T4, RM4-5, 1:500 dilution, BD Biosciences), CD8a FITC (clone 53-6.7, 1:500 dilution, BD Biosciences) and CD25 PE (PC61, 1:500 dilution, BD Biosciences). The gating strategy was: Thy1.2 + /TCRβ int /CD4 + /CD8 + for DP cells and Thy1.2 + /TCRβ low /CD4 − /CD8 − /CD25 + for DN2/3 cells. 3D DNA FISH and immuno-FISH 3D DNA FISH and combined DNA FISH-immunofluorescence for γ-H2AX (immuno-FISH) were carried out on T cells adhered to poly- L lysine-coated coverslips, as previously described [50] , [54] . Briefly, cells were fixed with 2% paraformaldehyde/PBS (pH 7–7.4) for 10 min at room temperature (RT) and permeabilized for 5 min with 0.4% Triton/PBS on ice. After 30 min of blocking in 2.5% BSA/10% normal goat serum/0.1% Tween-20/PBS, cells were sequentially incubated with a primary antibody against phosphorylated serine-139 of H2AX (γ-H2AX; Millipore) and a secondary goat-anti-mouse antibody (Alexa Fluor 488 or 555; Invitrogen) for 1 h each at RT. Cells were then post-fixed in 2% paraformaldehyde/PBS for 10 min at RT, incubated with 0.1 mg ml −1 RNaseA for 30 min at 37 °C and permeabilized in 0.7% Triton X-100/0.1 M HCl for 10 min on ice. Cells were then denatured with 50% formamide/2 × SSC (pH 7–7.4) for 30 min at 80 °C and hybridized overnight with the probes at 37 °C. The next day, cells were rinsed three times in 50% formamide/2 × SSC and three times in 2 × SSC at 37 °C for 5 min each. Finally, slides were mounted in ProLong Gold (Invitrogen) containing 1.5 μg ml −1 4',6-diamidino-2-phenylindole (DAPI). Probes BAC probes RP23-255N13 (3′α Tcra ), RP23-304L21 (5′α Tcra ), CT7-34H6 (3′ Igh ), RP24-386J17 (5′ Igh ), RP24-289O10 ( Hmgb1 ), RP24-358H24 ( Gapdh ), RP24-342A2 ( Lat ), RP23-410N16 ( Cd3g ), RP24-277H9 ( Ly6d ) and RP23-137H17 ( Satb1 ) were directly labelled by nick translation with ChromaTide Alexa Fluor 488 or 594-5-UTP (Molecular Probes) or Cy3- or Cy5-dUTP (Fisher). For one coverslip, 0.5 μg of nick-translation product was precipitated and resuspended in 10 μl of hybridization buffer (50% formamide/20% dextran sulphate/5 × Denhardt’s solution), denatured for 5 min at 95 °C and pre-annealed for 45 min at 37 °C before overnight hybridization with cells. XCyting Mouse Chromosome 14 (Texas-red) and 12 (FITC) paints (Metasystems) were prepared separately following the supplier’s instructions. Paint and BAC probes were combined just before overnight hybridization. Confocal microscopy and analysis 3D images were acquired by confocal microscopy on a Leica SP5 Acousto-Optical Beam Splitter system. Optical sections separated by 0.3 μm were collected, and stacks were analysed using Image J software. Alleles were defined as associated with γ-H2AX if the BAC signals and immunofluorescence foci were at least partially overlapped (at least one pixel of colocalization). Alleles were considered as located at PCH when BAC signals were adjacent or overlapping with a γ-satellite signal (no pixel in between the edges of the BAC and γ-satellite signals). Distances from the loci to their chromosome territories (higher-order looping) were measured from the centre of mass of the BAC signal to the closest edge of the chromosome paint. Distances between alleles or loci were measured between the centre of mass of each BAC signal. Statistical analyses The statistical tests were applied to combined data sets from repeated experiments. Supplementary Tables display individual experiments to show the low level of variation between the repeats. Statistical analyses were performed using a two-tail Fisher’s exact test: P -values ≤5.00e-2 ( a =0.05) were taken to be significant (1.00e-2≤ P ≤5.00e-2, *significant; 1.00e-3≤ P ≤1.00e-2, **very significant; and P <1.00e-3, ***highly significant). Circularized chromosome conformation capture (4C-seq) 4C-seq and domainogram analyses were performed as previously described [35] , [40] , [55] . Fixation and cell lysis: A total of 10 7 cells were resuspended in 5 ml PBS-10% FBS and fixed in 5 ml 4% formaldehyde-10% FBS for 10 min at RT (tumbling). A volume of 1.425 ml of 1 M glycine was added to quench crosslinking, and tubes were put on ice for 2 min. After 8-min centrifugation at 1,300 r.p.m. at 4 °C, pellets were resuspended in 1 ml cold ‘lysis buffer’ (50 mM Tris. pH 7.5, 150 mM NaCl, 5 mM EDTA, 0.5% NP-40, 1% Triton X-100 and 1 tablet mini complete) and incubated for 20 min on ice. After 5-min centrifugation at 1,800 r.p.m. at 4 °C, pellets were resuspended in 360 μl sterile water (or stored at − 80 °C). Hin dIII digestion : Nuclei were incubated for 1 h at 37 °C with 60 μl 10 × restriction buffer B and 15 μl 10% SDS (shaking). A concentration of 150 μl of 10% Triton X-100 were added, and nuclei were incubated for 1 h at 37 °C (shaking). In all, 5 μl of the sample was taken as the ‘undigested control’. Nuclei were incubated overnight at 37 °C with 400 U of Hin dIII restriction enzyme. Fresh enzyme was added for 6 more hours during the day. ‘Undigested’ and ‘digested’ controls (5 μl) were incubated in 90 μl Tris pH7.5 and 5 μl 10 mg ml −1 proteinase K for 2 h at 65 °C, DNA was extracted with 100 μl phenol-chloroform and the water phase was loaded on a 0.6% agarose gel. The Hin dIII enzyme was inactivated by adding 80 μl 10% SDS and incubating at 37 °C for 30 min. Ligation : Samples were transferred into 15 ml falcons and incubated with 4860 μl sterile water, 700 μl 10 × ligation buffer and 750 μl 10% Triton X-100 for 1 h at 37 °C (shaking). Ligases (50 U) were added and incubated overnight at 16 °C. A total of 100 μl of the sample was taken as the ‘ligated control’, tested as above (5 μl of 10 mg ml −1 proteinase K for 2 h at 65 °C and phenol extraction) and compared with the ‘digested control’ on a 0.6% agarose gel. De-crosslinking and precipitation : De-crosslinking was performed by adding 30 μl of 10 mg ml −1 proteinase K for 4 h at 65 °C. After 45-min incubation in 30 μl RNase A (10 mg ml −1 ) at 37 °C, DNA was phenol-extracted and ethanol-precipitated and resuspended in 150 μl 10 mM Tris pH 7.5. Dpn II digestion : Hin dIII-ligated 3C template was digested overnight at 37 °C with Dpn II (50 μl 10 × restriction buffer, 50 U Dpn II and 300 μl sterile water). Dpn II was inactivated at 65 °C for 30 min. Ligation and precipitation : DNA was ligated overnight at 16 °C in 12 ml sterile water, 1.4 ml ligation buffer and 100 U ligase. Ligation products were phenol-extracted and ethanol-precipitated using glycogen as a carrier (20 mg ml −1 ), and they were resuspended in 75 μl 10 mM Tris pH 7.5. Samples were purified using Illustra GFX PCR DNA and Gel Band Purification Kit (GE Healthcare). PCR reaction and sequencing : Specific primers for the Tcra Eα enhancer were Hin dIII 5′-AGACAGACCCTGCGAAGCTT-3′ and Dpn II 5′-TAAGACTGGACCCACAG-3′. The Illumina-specified adapters for Illumina GAIIx sequencing were included at the 5′ end of each primer. PCR reactions were performed using the Expand Long Template PCR system (Roche), and PCR conditions were as following: 94 °C for 2 min; 30 cycles of 94 °C for 1 min, 55 °C for 1 min and 68 °C for 3 min; followed by a final step of 68 °C for 7 min. The 4C library was sequenced on an Illumina GAIIx single-read 72-cycle run. 4C-seq analysis : The 54-bp single-end reads were aligned to a library of 40-bp flanking regions of Hin dIII restriction sites, on the mouse genome sequence (build mm9). The alignment was performed using Maq software ( http://maq.sourceforge.net/ ) with a quality threshold of 150. We kept the distinction between the upstream and downstream flanking region of each Hin dIII site. We segmented the genome according to the Hin dIII restriction sites and removed those segments consisting of two consecutive Hin dIII restriction sites that did not contain a Dpn II restriction site. Domainogram analysis : We followed the analytical steps described previously [38] , using the genomic regions enclosed between two contiguous Hin dIII sites. We then used windows of increasing size extending up to 30 Hin dIII sites. We computed and analysed scores in each window size as follows: first, we scored each pair of contiguous Hin dIII sites (defined as Q ( x )=(rank( x )−0.5)/ N , where Q is a quantile score of Hin dIII sites ( x ) and N is the total number of these sites). The Q i-values are calculated in a global manner for the whole genome, with the bait chromosome analysed separately. We transformed the combination of scores within each window to a form that was amenable to applying Fisher’s approach for combining independent tests of significance. The range of colours in the domainograms represents the intensity of these scores. See Supplementary Table S4 for details. Chromatin immunoprecipitation sequencing Chromatin immunoprecipitation sequencing (ChIP-seq) preparation was carried out as previously described [56] , and ChIP-seq analysis was performed using the Qeseq algorithm [57] (details were provided in Chaumeil et al. [40] ). Cell fixation and lysis : A total of 1–5 × 10 6 cells were fixed in 1% formaldehyde for 10 min at RT and lysed in 15 mM Tris pH 7.5, 60 mM KCl, 15 mM NaCl, 15 mM MgCl 2 , 1 mM CaCl 2 , 250 mM sucrose and 0.3% NP-40 for 10 min at 4 °C. Nuclei were isolated by centrifugation and washed once in ‘digest buffer’ (10 mM NaCl, 10 mM Tris-HCl, pH 7.5, 3 mM MgCl 2 , 1 mM CaCl 2 and 0.1 mM phenylmethylsulphonyl fluoride). Chromatin preparation : Mononucleosomal particles were generated using Micrococcal nuclease (USB) in ‘digest buffer’ (reaction stopped with 20 mM EDTA). Nuclei were then lysed in ‘nucleus lysis’ buffer (50 mM Tris-HCl (pH 8.0), 10 mM EDTA (pH 8.0) and 1% SDS) and sonicated (2.5 min total; Bioruptor (Diagenode)). Chromatin was pre-cleared by addition of nine volumes of ‘IP dilution’ buffer (0.01% SDS, 1.1% Triton X-100, 1.2 mM EDTA (pH 8.0), 16.7 mM Tris-HCl (pH 8.0) and 167 mM NaCl) and magnetic Dynal beads. Chromatin (1%) was saved as ‘input’. Chromatin immunoprecipitation : Antibodies (H3K4me3; Active Motif and H3K9ac; Abcam) and beads were incubated together for 4 h in ‘IP dilution’ buffer, before overnight incubation with the chromatin at 4 °C, while rotating. The complexes bound on the beads were then washed in buffers with increasing salt concentration (‘wash A’: 20 mM Tris-HCl pH 8, 150 mM NaCl, 2 mM EDTA, 1% w/v Triton and 0.1% w/v SDS; ‘wash B’: 20 mM Tris-HCl, pH 8.0, 500 mM NaCl, 2 mM EDTA, 1% w/v Triton and 0.1% w/v SDS; ‘wash C’: 10 mM Tris-HCl, pH8.0, 250 mM LiCl, 1 mM EDTA, 1% w/v Nonidet P-40 and 1% w/v deoxycholic acid) and twice with TE buffer. The bound chromatin was cleaned using proteinase K and incubated at 65 °C overnight, and DNA was phenol-extracted and ethanol-precipitated. ChIP-seq libraries and sequencing : ChIP-seq libraries were generated using standard Illumina kit protocol. Truseq adapters were added, and the libraries were PCR-amplified. Size selection was performed using E-gel electrophoresis system by Invitrogen. Cluster amplification and 36-nucleotide single-end sequencing on an Illumina Genome Analyzer II were performed following the manufacturer’s instructions. ChIP-seq analysis : Reads were aligned with Bowtie 0.12.7 software to the reference mouse genome (mouse assembly NCBI mm9), using the following command line option-best-all –m1 –n2 (reads that align uniquely in the best alignment stratum, allowing up to two mismatches). See Supplementary Table S5 for details. Western blotting Cells were incubated in lysing buffer (0.2% sodium dodecyl sulphate and 100 mM Tris-HCL) at 16,000 cells per μl for 5 min at 95 °C and treated with Bensonaze nuclease (0.05 U μl −1 ) for removal of nucleic acids for 5 min at RT. Protein extracts were denatured and reduced in 1 × Nupage sample LDS and 1 × Nupage sample reducing agent (Life Technologies) for 5 min at 95 °C before the equivalent of 2 × 10 5 cells per lane was loaded. Membranes were blocked in PBS with 5% milk and 0.1% Tween and incubated with the following primary antibodies in 5% milk and 0.1% Tween: ATM (MAT3-4G10/8, 1/4,000; Abcam) and γ-Tubulin (clone GTU-88; 1/5,000; Sigma), which was used as a loading control. Blots were developed with enhanced chemiluminescence (Pierce). How to cite this article: Chaumeil, J. et al. The RAG2 C-terminus and ATM protect genome integrity by controlling antigen receptor gene cleavage. Nat. Commun. 4:2231 doi: 10.1038/ncomms3231 (2013).